Rapamycin reverses impaired social interaction in mouse models of tuberous sclerosis complex Impairment of reciprocal social interaction is a core symptom of autism spectrum disorder. Genetic disorders frequently accompany autism spectrum disorder, such as tuberous sclerosis complex caused by haploinsufficiency of the TSC1 and TSC2 genes. Accumulating evidence implicates a relationship between autism spectrum disorder and signal transduction that involves tuberous sclerosis complex 1, tuberous sclerosis complex 2 and mammalian target of rapamycin. Here we show behavioural abnormalities relevant to autism spectrum disorder and their recovery by the mammalian target of rapamycin inhibitor rapamycin in mouse models of tuberous sclerosis complex. In Tsc2 +/− mice, we find enhanced transcription of multiple genes involved in mammalian target of rapamycin signalling, which is dependent on activated mammalian target of rapamycin signalling with a minimal influence of Akt. The findings indicate a crucial role of mammalian target of rapamycin signalling in deficient social behaviour in mouse models of tuberous sclerosis complex, supporting the notion that mammalian target of rapamycin inhibitors may be useful for the pharmacological treatment of autism spectrum disorder associated with tuberous sclerosis complex and other conditions that result from dysregulated mammalian target of rapamycin signalling. Autism spectrum disorder (ASD) affects >1% of the general population [1] . It consists of impaired social interaction, impaired communication and repetitive and restricted behaviours and interests [2] , among which impaired social interaction is most essential [3] , [4] . The significance of genetic factors in the aetiology of ASD is emphasized by the high heritability of ASD in monozygotic twins [5] and single-gene defects and copy number variations in individuals with ASD [6] , [7] , [8] . However, advances in ASD genetics have not yet provided effective therapies against the social impairment associated with ASD. The pharmacological treatment of ASD is largely limited to the symptomatic level, targeting irritability, aggression and agitation [9] . Tuberous sclerosis complex (TSC) is an autosomal dominant disorder caused by mutations in either the TSC1 or TSC2 gene [10] , [11] . The neurological phenotype of TSC is divided into pathological and functional abrration. Pathological abnormalities include astrocytomas and cortical tubers, a malformative lesion occurring in almost all individuals with TSC. The functional abnormalities are diverse (for example, epilepsy syndromes, such as infantile spasms and intellectual disability) [12] . At the molecular level, the protein products of TSC1 , hamartin and TSC2 , tuberin, form a heterodimer that inhibits Ras homologue enriched in the brain (Rheb) [13] , a small G protein that activates mammalian target of rapamycin (mTOR) complex 1 (mTORC1). Heterozygous defects in either TSC gene cause excessive mTOR activation, which in turn provokes abnormal acceleration of important cellular events, such as cell growth and proliferation [13] , [14] . TSC is notable for its high association with ASD. Approximately half of the patients with TSC meet the criteria for ASD [15] , [16] , [17] , [18] , and 1–4% of ASD cases are attributable to TSC [6] , [8] . TSC is thus one of the most frequent causes of syndromic ASD [6] , [8] . The close relationship between TSC and ASD has been explained on the basis of the direct consequence of deficient hamartin and tuberin, resulting in uninhibited mTOR signalling in the brain [19] , [20] . This hypothesis is supported by the following epidemiological observations. The sex ratio of individuals with TSC-related ASD is equal, in contrast to the skewed male susceptibility to ASD in general [16] , [17] . ASD occurs in 20% of TSC patients with normal intelligence, far more frequent than in the general population [17] . However, epidemiological links between ASD and cortical tubers or epilepsy have been controversial, questioning whether those complications have pathogenetic roles [16] , [17] , [18] , [21] , [22] . To elucidate the significance of uninhibited mTOR signalling in ASD associated with TSC, eliminating the confounding effects of the neurological complications mentioned above is necessary, which is nearly impossible in the clinical setting. Rodents that harbour a defect in the Tsc1 or Tsc2 gene have been extensively investigated [23] , [24] , [25] , [26] . Homozygous mutants are embryonically lethal, and heterozygotes develop tumours in various organs [23] , [24] . Intriguingly, mutant animals show neurological manifestations that are partially distinct from human TSC. Cortical tubers are absent in Tsc1 +/− and Tsc2 +/− rodents [25] , [27] , with exceptional occurrence in Eker rats [28] , a strain with a spontaneous mutation in the Tsc2 gene. No report has described epileptic seizures in Tsc1 +/− and Tsc2 +/− rodents, whether spontaneous or induced by external stimuli. Nonetheless, Tsc1 +/− and Tsc2 +/− mice exhibit learning and memory deficits [27] , [29] . The mTOR inhibitor rapamycin reverses learning deficits in Tsc2 +/− mice [29] , suggesting that pharmacological therapy of cognitive impairment in TSC should be directed towards mTOR inhibition [14] , [19] , [20] . Rodent models of TSC, which basically lack cortical tubers and epilepsy, appear to be appropriate for examining the causal role of mTOR signalling in ASD. However, autism-like behavioural abnormalities have been noticed in female Tsc1 +/− mice [27] and male Eker rats [30] , although not in Tsc2 +/− mice [29] , [31] . Systematic evaluation of ASD associated with TSC requires behavioural and molecular investigations on both Tsc1 +/− and Tsc2 +/− mice using the same methods. In the present study, we examined Tsc1 +/− and Tsc2 +/− mice of both sexes using the same testing protocol and observed deficient social behaviours relevant to core disabilities in ASD. Rapamycin reversed the behavioural abnormalities in Tsc1 +/− and Tsc2 +/− mice. In the brains of Tsc2 +/− mice, mRNA expression and the phosphorylation of proteins related to the mTOR signalling pathway were altered and reversed by rapamycin. Given these findings, mTOR inhibitors may be useful for ASD associated with mTOR activation, even in adulthood. Deficient social interaction in Tsc mutant mice We first examined the mice using the social interaction test. Tsc1 +/− and Tsc2 +/− mice spent a shorter time engaged in active interaction (that is, exploring a novel mouse) than wild-type (WT) littermates ( P <0.0001 ( Tsc1 ), P =0.0010 ( Tsc2 ) by two-way analysis of variance (ANOVA); Fig. 1a , Supplementary Movie 1 and 2 ). The reduction was not dependent on sex ( P =0.80 ( Tsc1 ), P =0.32 ( Tsc2 )) and remained significant in all subgroups segregated by mouse strain and sex ( P <0.0001 (male Tsc1 ), P =0.0099 (female Tsc1 ), P =0.018 (male Tsc2 ), P= 0.025 (female Tsc2 ) by two-tailed t -test). Tsc1 +/− and Tsc2 +/− mice also exhibited an increase in rearing behaviour ( P <0.0001 [ Tsc1 ], P <0.0001 [ Tsc2 ] by two-way ANOVA; Fig. 1b ). The difference was independent of sex ( P =1.0 ( Tsc1 ), P =0.14 ( Tsc2 )) and persisted in every subgroup ( P =0.0047 (male Tsc1 ), P =0.0020 (female Tsc1 ), P =0.0021 (male Tsc2 ), P =0.0072 (female Tsc2 ) by two-tailed t -test). In the tube test, which examines social dominance, Tsc1 +/− and Tsc2 +/− mice and WT littermates won equally ( P =0.35 (male Tsc1 ), P =0.43 (female Tsc1 ), P =0.42 (male Tsc2 ), P =0.50 (female Tsc2 ); Fig. 1c , Supplementary Table S1 ). These results indicate that deficient social interaction in Tsc mutant mice is not derived from altered social dominance. 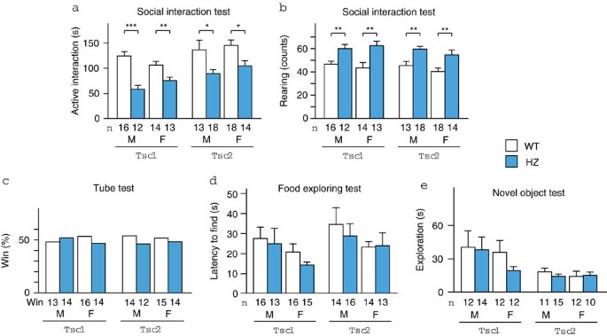Figure 1: Behavioural phenotype ofTsc1+/−andTsc2+/−mice. (a) Active interaction time in the 10 min social interaction test. (b) Counts of rearing behaviour during the test. The data were compared between WT and heterozygous (HZ) mice. (c) The tube test showed no difference in social dominance between WT and HZ mice. (d) Time elapsed to find buried food in the food exploration test. (e) Total duration of exploring the object in the novel object test. F, female; M, male. The number of mice tested is shown in each panel. Error bars indicate s.e.m. *P<0.05, **P<0.01, ***P<0.001 (two-tailedt-test). Figure 1: Behavioural phenotype of Tsc1 +/− and Tsc2 +/− mice. ( a ) Active interaction time in the 10 min social interaction test. ( b ) Counts of rearing behaviour during the test. The data were compared between WT and heterozygous (HZ) mice. ( c ) The tube test showed no difference in social dominance between WT and HZ mice. ( d ) Time elapsed to find buried food in the food exploration test. ( e ) Total duration of exploring the object in the novel object test. F, female; M, male. The number of mice tested is shown in each panel. Error bars indicate s.e.m. * P <0.05, ** P <0.01, *** P <0.001 (two-tailed t -test). Full size image We tested olfaction and exploratory behaviour, deficits of which could interfere with social interaction. Tsc1 +/− and Tsc2 +/− mice exhibited normal olfaction in the food exploration test compared with WT littermates (genotype: P =0.40 ( Tsc1 ), P =0.68 ( Tsc2 ); sex: P =0.11 ( Tsc1 ), P =0.22 ( Tsc2 ); Fig. 1d ). Exploration towards an inanimate object was unaffected by genotype and sex (genotype: P =0.43 ( Tsc1 ), P =0.66 ( Tsc2 ); sex: P =0.38 ( Tsc1 ), P =0.65 ( Tsc2 ); Fig. 1e ). Altogether, Tsc mutant mice appeared to exhibit impaired social interaction because they were specifically less interested in novel mice. Intact motor and sensory function in Tsc mutant mice We checked general and neurologic conditions and motor and sensory function. No overt abnormalities were found with regard to general condition, neurologic reflexes or body weight in Tsc1 +/− and Tsc2 +/− mice ( Supplementary Tables S2 and S3 ). The mutant mice exhibited no motor deficits in the open-field test (genotype: P =0.92 ( Tsc1 ), P =0.26 ( Tsc2 ); sex: P =0.77 ( Tsc1 ), P =0.14 ( Tsc2 ); Fig. 2a ), pole test (genotype: P =0.29 ( Tsc1 ), P =0.63 ( Tsc2 ); sex: P =0.97 ( Tsc1 ), P =0.28 ( Tsc2 ); Fig. 2b ) or rotarod test (time course: P <0.0001 ( Tsc1 ), P <0.0001 ( Tsc2 ) by three-way mixed-design ANOVA; genotype: P =0.21 ( Tsc1 ), P =0.49 ( Tsc2 ); sex: P =0.67 ( Tsc1 ), P =0.074 ( Tsc2 ); Fig. 2c ). Pain sensitivity in the hot plate test was similar between genotype and sex (genotype: P =0.66 ( Tsc1 ), P =0.23 ( Tsc2 ); sex: P =0.46 ( Tsc1 ), P =0.37 ( Tsc2 ); Fig. 2e ). In the tail flick test, male Tsc1 mice had longer latencies than female Tsc1 mice ( P =0.0045 by two-way ANOVA), whereas male and female Tsc2 mice responded similarly ( P =0.18; Fig. 2f ). Genotype did not affect these results ( P =0.65 ( Tsc1 ), P =0.82 ( Tsc2 )). These results indicate the absence of significant abnormalities in motor and sensory function in Tsc1 +/− and Tsc2 +/− mice. 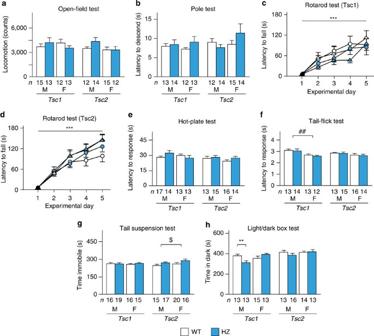Figure 2: Motor ability and sensory function inTsc1+/−andTsc2+/−mice. (a) Locomotor activity for 120 min. (b) Time to descend in the pole test. (c) Latency to fall in the rotarod test inTsc1+/−mice (open circles, male WT,n=10; blue circles, male HZ,n=10; open triangles, female WT,n=10; blue triangles, female HZ,n=11). (d) Latency to fall in the rotarod test inTsc2+/−mice (open circles, male WT,n=14; blue circles, male HZ,n=12; open triangles, female WT,n=10; blue triangles, female HZ,n=11). (e) Latency to lick the hindpaws or jump in the hot-plate test. (f) Latency to response in the tail-flick test. (g) Immobility time in the tail suspension test. (h) Time in the dark chamber in the light/dark box test. F, female; M, male. The number of mice tested is shown in each panel. Error bars indicate s.e.m. **P<0.01 (genotype effect; two-tailedt-test); ***P<0.001 (time-course effect; three-way mixed-design ANOVA);##P<0.01 (sex effect; two-way ANOVA);$P<0.05 (genotype effect; two-way ANOVA). Figure 2: Motor ability and sensory function in Tsc1 +/− and Tsc2 +/− mice. ( a ) Locomotor activity for 120 min. ( b ) Time to descend in the pole test. ( c ) Latency to fall in the rotarod test in Tsc1 +/− mice (open circles, male WT, n =10; blue circles, male HZ, n =10; open triangles, female WT, n =10; blue triangles, female HZ, n =11). ( d ) Latency to fall in the rotarod test in Tsc2 +/− mice (open circles, male WT, n =14; blue circles, male HZ, n =12; open triangles, female WT, n =10; blue triangles, female HZ, n =11). ( e ) Latency to lick the hindpaws or jump in the hot-plate test. ( f ) Latency to response in the tail-flick test. ( g ) Immobility time in the tail suspension test. ( h ) Time in the dark chamber in the light/dark box test. F, female; M, male. The number of mice tested is shown in each panel. Error bars indicate s.e.m. ** P <0.01 (genotype effect; two-tailed t -test); *** P <0.001 (time-course effect; three-way mixed-design ANOVA); ## P <0.01 (sex effect; two-way ANOVA); $ P <0.05 (genotype effect; two-way ANOVA). Full size image The mice were then analysed for depression and anxiety because these two conditions are commonly found in TSC-related ASD [16] , [17] . In the tail suspension test, immobility time in Tsc2 +/− mice was longer than in WT littermates ( P =0.63 ( Tsc1 ), P =0.044 ( Tsc2 ) by two-way ANOVA; Fig. 2g ), whereas no difference was observed for sex ( P =0.87 ( Tsc1 ), P =0.12 ( Tsc2 )). This finding may correspond to a more severe TSC2 mutation phenotype [16] , [23] , [24] , [32] , [33] . In the light/dark box test, the time spent in the dark compartment was not different for genotype and sex (genotype: P =0.41 ( Tsc1 ), P =0.64 ( Tsc2 ); sex: P =0.17 ( Tsc1 ), P =0.35 ( Tsc2 ); Fig. 2h ). However, a significant genotype × sex interaction was found in Tsc1 mice ( P =0.0059), and male Tsc1 +/− mice spent less time in the dark chamber than WT mice ( P =0.0099 by two-tailed t -test), suggesting low anxiety in male Tsc1 +/− mice. Recovered social deficits in Tsc mutant mice by rapamycin The effects of mTOR inhibition on reduced social interaction were then examined using adult heterozygotes. Active interaction in Tsc1 +/− and Tsc2 +/− mice responded to rapamycin treatment ( P =0.0012 ( Tsc1 ), P =0.0023 ( Tsc2 ) by one-way ANOVA; Fig. 3a ), whereas WT mice did not respond to this treatment ( P =0.80 ( Tsc1 ), P =0.98 ( Tsc2 )). In both heterozygotes, rapamycin extended the time of active interaction at doses of 5 and 10 mg kg −1 ( P <0.05 by Dunette post hoc test; Supplementary Movie 3 ), although 2 mg kg −1 was ineffective ( P >0.05). When the genotypes were compared, the mutant mice displayed a reduction of active interaction following treatment with vehicle ( P =0.022 ( Tsc1 ), P =0.014 ( Tsc2 ) by two-tailed t -test) and 2 mg kg −1 rapamycin ( P =0.028 ( Tsc1 ), P =0.028 ( Tsc2 ) by two-tailed t -test). Active interaction time was equal between genotypes after rapamycin injections of 5 mg kg −1 ( P =0.50 ( Tsc1 ), P =1.0 ( Tsc2 )) and 10 mg kg −1 ( P =0.51 ( Tsc1 ), P =0.86 ( Tsc2 )). These results indicate that rapamycin recovered social interaction specifically in Tsc1 +/− and Tsc2 +/− mice. 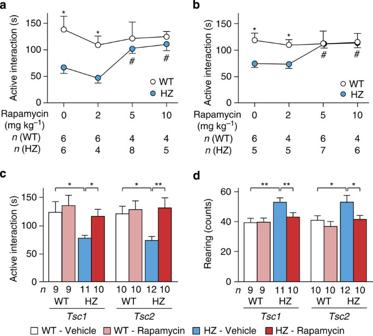Figure 3: Effects of rapamycin on social interaction and rearing inTsc1+/−andTsc2+/−mice. (a) Active interaction time inTsc1+/−mice treated with different doses of rapamycin. (b) Active interaction time inTsc2+/−mice treated similarly. (c) Active interaction time inTsc1+/−andTsc2+/−mice treated with 5 mg kg−1rapamycin. (d) Counts of rearing behaviour inTsc1+/−andTsc2+/−mice during the test. The mice that were used incanddwere independent of those used in (aandb). Error bars indicate s.e.m. *P<0.05, **P<0.01 (two-tailedt-test);#P<0.05 (dose effect; Dunnett’spost hoctest). Figure 3: Effects of rapamycin on social interaction and rearing in Tsc1 +/− and Tsc2 +/− mice. ( a ) Active interaction time in Tsc1 +/− mice treated with different doses of rapamycin. ( b ) Active interaction time in Tsc2 +/− mice treated similarly. ( c ) Active interaction time in Tsc1 +/− and Tsc2 +/− mice treated with 5 mg kg −1 rapamycin. ( d ) Counts of rearing behaviour in Tsc1 +/− and Tsc2 +/− mice during the test. The mice that were used in c and d were independent of those used in ( a and b ). Error bars indicate s.e.m. * P <0.05, ** P <0.01 (two-tailed t -test); # P <0.05 (dose effect; Dunnett’s post hoc test). Full size image Independent groups of mice were then examined for active interaction and rearing behaviour after treatment with 5 mg kg −1 rapamycin. Tsc1 +/− and Tsc2 +/− mice that received vehicle exhibited a decrease in active interaction ( P =0.034 ( Tsc1 ), P =0.014 ( Tsc2 ) by two-tailed t -test; Fig. 3c ) and increase in rearing behaviour ( P =0.010 ( Tsc1 ), P =0.024 ( Tsc2 ) by two-tailed t -test; Fig. 3d ). Rapamycin treatment in the heterozygotes normalized active interaction ( P =0.018 ( Tsc1 ), P =0.0092 ( Tsc2 ) by two-tailed t -test; Fig. 3c ) and attenuated rearing behaviour ( P =0.0074 ( Tsc1 ), P =0.027 ( Tsc2 ) by two-tailed t -test; Fig. 3d ). WT mice did not respond to rapamycin with regard to active interaction ( P =0.67 ( Tsc1 ), P =0.74 ( Tsc2 ); Fig. 3c ), rearing behaviour ( P =1.0 ( Tsc1 ), P =0.34 ( Tsc2 ); Fig. 3d ), or locomotor activity ( Tsc1 : 3,823±489 versus 3,176±385, P =0.31, Tsc2 : 3,223±283 versus 3,087±286, P =0.74; mean±s.e.m.). Altered gene and protein expressions in Tsc2 +/− mice The above findings suggest that haploinsufficiency of the Tsc1 or Tsc2 gene leads to uninhibited mTOR signalling and impaired social interaction. To determine the pathogenetic role of mTOR signalling, we analysed the brains from Tsc2 +/− mice because Tsc2 mutations result in more severe phenotypic manifestations in mice [23] , [24] , [33] and humans [16] , [32] . First, genes in the TSC-mTOR pathway were screened for mRNA expression intensity ( Fig. 4a ). In Tsc2 +/− mice, Tsc2 mRNA intensity was lower than in WT animals ( P =0.0011 by two-tailed t -test) and further decreased by rapamycin ( P =0.039 by two-tailed t -test; Fig. 4b ). Tsc1 mRNA intensity was elevated ( P =0.049 by two-tailed t -test), but its response to rapamycin was marginal ( P =0.061; Fig. 4b ). Among the genes upstream of Tsc1 and Tsc2 , Gsk3b (that is, the gene that encodes for GSK3β) and Mapk1 (that is, the gene that encodes for ERK2) showed higher mRNA intensities in Tsc2 +/− mice ( P =0.0081 ( Gsk3b ), P =0.038 ( Mapk1 ) by two-tailed t -test), and rapamycin reversed them ( P =0.023( Gsk3b ), P =0.016 [ Mapk1 ) by two-tailed t -test; Fig. 4b ). No changes were noticed in the mRNA levels of the other genes ( Supplementary Fig. S1 ). Among the genes downstream of mTORC1, Ulk1 , Igbp1 , Rps6 (that is, the gene that encodes for S6) and Eef2k were increased in Tsc2 +/− mice ( P =0.039 ( Ulk1 ), P =0.043 ( Igbp1 ), P =0.036 ( Rps6 ) , P =0.034 ( Eef2k ) by two-tailed t -test; Fig. 4b ). Rapamycin suppressed the expression of Ulk1 and Eef2k ( P =0.026 ( Ulk1 ), P =0.049 ( Eef2k ) by two-tailed t -test; Fig. 4b ) but not Igbp1 ( P =0.10) or Rps6 ( P =0.27; Supplementary Fig. S2 ). Among the components of mTORC1 and mTORC2, Deptor mRNA expression was enhanced in Tsc2 +/− mice ( P =0.0021 by two-tailed t -test) and normalized by rapamycin ( P =0.033 by two-tailed t -test; Fig. 4b ). The transcription of the other genes illustrated in Fig. 4a remained unaltered in Tsc2 +/− brains ( Supplementary Fig. S2 and S3 ). 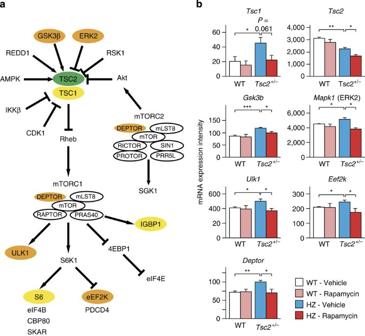Figure 4: Transcription of the genes associated with mTOR signalling. (a) mTOR signalling pathway in which mRNA expression was screened. Coloured genes represent the following: orange (genes whose levels showed a significant increase inTsc2+/−mice and significant decrease following rapamycin treatment), yellow (genes whose levels showed a significant increase inTsc2+/−mice and no reversal following rapamycin treatment), green (gene whose levels showed a significant decrease inTsc2+/−mice and a further decline following rapamycin treatment). (b) Expression intensities of the genes that showed a significant change and response to rapamycin inTsc2+/−mice (n=4 for each group segregated by genotype and treatment). Error bars indicate s.e.m. *P<0.05, **P<0.01, ***P<0.001 (two-tailedt-test). Figure 4: Transcription of the genes associated with mTOR signalling. ( a ) mTOR signalling pathway in which mRNA expression was screened. Coloured genes represent the following: orange (genes whose levels showed a significant increase in Tsc2 +/− mice and significant decrease following rapamycin treatment), yellow (genes whose levels showed a significant increase in Tsc2 +/− mice and no reversal following rapamycin treatment), green (gene whose levels showed a significant decrease in Tsc2 +/− mice and a further decline following rapamycin treatment). ( b ) Expression intensities of the genes that showed a significant change and response to rapamycin in Tsc2 +/− mice ( n =4 for each group segregated by genotype and treatment). Error bars indicate s.e.m. * P <0.05, ** P <0.01, *** P <0.001 (two-tailed t -test). Full size image The seven genes (that is, Tsc1 , Tsc2 , Deptor , Ulk1 , Eef2k , Gsk3b and Mapk1 ) were then quantified using real-time PCR. In Tsc2 +/− mice, the level of Tsc2 mRNA was reduced to two-thirds of the levels in WT mice ( P =0.0041 by two-tailed t -test) and insensitive to rapamycin ( Supplementary Table S4 ). Tsc1 mRNA levels nearly doubled ( P =0.0023 by two-tailed t -test) and returned to WT levels with rapamycin treatment ( P =0.00066 by two-tailed t -test; Supplementary Table S4 ). Only slight changes in mRNA levels were noticed for Gsk3b , Mapk1 , Deptor and Ulk1 ( Supplementary Table S4 ). We did not obtain measurable transcripts for the Eef2k gene. Finally, the status of the Tsc-mTOR signalling pathway followed by rapamycin treatment was examined at the protein level. In Tsc2 +/− mice, mTOR activation was reflected by an elevation of phospho-S6K levels ( P =0.012 by two-tailed t -test; Fig. 5a ). Two doses of rapamycin effectively suppressed S6K phosphorylation ( P =0.026 by two-tailed t -test; Fig. 5a ), whereas the treatment did not change total S6K levels ( Supplementary Table S5 ). A mild decrease in tuberin was noticed in Tsc2 +/− brains ( P =0.023 by two-way ANOVA), which was not rescued by rapamycin ( P =0.87; Fig. 5a ). The obvious change in Tsc1 mRNA expression did not affect hamartin levels ( P =0.25 (genotype), P =0.40 (treatment); Fig. 5a ). We measured Akt phosphorylation because feedback inhibition of Akt by S6K [34] , [35] , [36] may modulate behaviour in Tsc2 +/− mice. Akt phosphorylation was mildly reduced in Tsc2 +/− mice ( P =0.024 by two-way ANOVA; Fig. 5a ) and unresponsive to rapamycin ( P =0.92; Fig. 5a ). Total Akt levels remained unchanged by Tsc2 haploinsufficiency and rapamycin ( Supplementary Table S5 ). 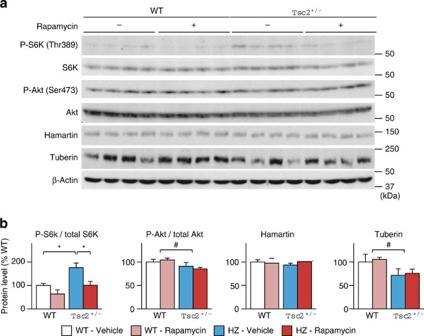Figure 5: Western blots of proteins associated with the mTOR signalling pathway. (a) Immunoblots for phospho- and total S6K, phospho- and total Akt, hamartin and tuberin. (b) Densitometric analysis of the four proteins (n=4 for each group segregated by genotype and treatment). Error bars indicate s.e.m. *P<0.05 (two-tailedt-test);#P<0.05 (genotype effect; two-way ANOVA). Figure 5: Western blots of proteins associated with the mTOR signalling pathway. ( a ) Immunoblots for phospho- and total S6K, phospho- and total Akt, hamartin and tuberin. ( b ) Densitometric analysis of the four proteins ( n =4 for each group segregated by genotype and treatment). Error bars indicate s.e.m. * P <0.05 (two-tailed t -test); # P <0.05 (genotype effect; two-way ANOVA). Full size image In the present study, we observed impaired social behaviour in Tsc1 +/− and Tsc2 +/− mice of both sexes. Moreover, the mTOR inhibitor rapamycin reversed the abnormality in adult heterozygotes. In Tsc2 +/− mice, the behavioural improvement was associated with inhibition of mTOR at the molecular level. These findings indicate that haploinsufficiency of the Tsc1 or Tsc2 gene causes social deficits via uninhibited mTOR signalling and that pharmacological inhibition of mTOR rescues social impairment in TSC, even in adulthood. Earlier studies have disagreed with regard to deficient social behaviours in rodent models of TSC, partially because either Tsc1 +/− or Tsc2 +/− mice were investigated or different tasks were applied in each study [27] , [29] , [30] , [31] . By analysing Tsc1 +/− and Tsc2 +/− mice in the same environment and using the same testing approach, we found that these mutant animals exhibit a reduction of active interaction in the social interaction test, a core behavioural deficit relevant to ASD in humans [3] , [4] and rodents [37] . This finding is consistent with the strong association between TSC and ASD [15] , [16] , [17] , [18] , [19] , [20] . In addition, the impairment was similar in magnitude between male and female heterozygotes, reflecting the equal sex ratio in human patients with TSC-related ASD [16] , [17] . The reduced social interaction was unlikely derived from aversion to social or non-social novelty because social dominance and novelty exploration were unchanged. The reduction mentioned above contrasts with unaltered sociability in Tsc2 +/− mice [29] , [31] , which may be attributable to different testing approaches. In this context, behavioural analyses of an Fmr1 knockout mouse model of Fragile X syndrome (FXS), another leading cause of syndromic ASD [6] , [8] , have also provided apparently conflicting data. The social recognition test revealed lower social interaction [38] , whereas the three-chambered social approach task did not find deficient sociability [39] . Assays that allow direct contact with novel animals may be more sensitive to the detection of social deficits in rodents, including Tsc1 +/− , Tsc2 +/− and Fmr1 knockout mice. The present study first found that mTOR inhibition normalized deficient social interaction in Tsc1 +/− and Tsc2 +/− mice. As reported previously, rapamycin rescued learning deficits in Tsc2 +/− mice [29] . Rapamycin also reduced seizure frequency and ameliorated histological abnormalities in mice that lacked the Tsc1 or Tsc2 gene in astrocytes [33] . Impaired social interaction in female Tsc1 +/− mice [27] and male Eker rats [30] , however, has not been investigated with regard to its treatment using mTOR inhibitors. Given that Tsc1 +/− and Tsc2 +/− mice lack cortical tubers and epileptic seizures [25] , [27] , the present research indicates that uninhibited mTOR that results from a mutation in the Tsc1 or Tsc2 gene directly disrupts social interaction. The above finding also highlights the usefulness of Tsc1 +/− and Tsc2 +/− mice as mouse models of pharmacologically treatable ASD. The effectiveness of rapamycin was demonstrated on one of the triad symptoms of ASD, impairment of reciprocal social interaction. Future research should focus on the remaining two components of ASD, impairment in communication and restrictive and repetitive behaviour. In the present study, we observed an increase in rearing behaviour in Tsc1 +/− and Tsc2 +/− mice, which also responded to rapamycin. Remaining unknown, however, is what this behaviour represents with regard to ASD. Generally, rearing behaviour is considered an exploratory or escape behaviour [40] , [41] . Its significance may vary depending on the species, strains and experimental conditions. Rearing behaviour is decreased in some rodent strains with social deficits [30] , [40] , [42] , whereas it is increased in others [43] . The behaviour may be stimulated by environmental stress. For example, BALB/cJ mice, an inbred strain that exhibits autism-like behaviour [40] , showed a marked increase in rearing behaviour after exposure to a rat [44] . Fmr1 knockout mice engaged in rearing and digging more than WT mice during a three-chambered social approach task [45] . These facts allow us to speculate that the environment in the social interaction test may have either heightened the interest of Tsc1 +/− and Tsc2 +/− mice in the overhead direction or prompted them to escape from the environment. The effectiveness of rapamycin on this behaviour indicates that the increase in rearing behaviour is caused by dysregulated mTOR signalling. Research is necessary to reveal the underlying mechanisms of rearing behaviour and its significance, particularly with regard to ASD. The disruption of Tsc1 or Tsc2 and subsequent hyperactivation of mTOR elicit several feedback responses. Particularly important is the feedback inhibition of Akt via S6K, a negative regulator of TSC2 [34] , [35] , [36] . Akt phosphorylation is elevated in mice with deletions in Pax6 [46] and Pten [47] , [48] . Impaired social interaction in these animals suggests the behavioural influence of Akt [42] , [47] , [48] . In Pten mutant mice, chronic treatment with rapamycin suppressed the phosphorylation of Akt and S6 and ameliorated the impairment in social interaction [48] . Thus, remaining to be solved was whether Akt, mTOR or both regulate social behaviour. In Tsc2 +/− mice given short-term treatment with rapamycin, the feedback suppression of Akt remained unchanged when S6K phosphorylation and social interaction returned to normal. Rapamycin restored behavioural abnormalities and mTOR signalling, suggesting that uninhibited mTOR signalling is chiefly responsible for the social deficits in mouse models of TSC. This strongly supports the ‘global regulator and integrator of a range of physiological processing (GRIPP) hypothesis’, in which mTOR activation produces cognitive impairments and neuropsychiatric conditions, such as ASD in TSC [19] , [20] . The present findings, in addition to earlier animal studies, will prompt clinical research on the pharmacotherapy of neuropsychiatric disorders, such as ASD, with mTOR inhibitors. Rapamycin improved a wide range of neurological derangements, learning deficits, epileptic seizures and neuronal abnormalities in mouse models of TSC [29] , [33] . In clinical trials of the mTOR inhibitors rapamycin and everolimus for TSC-associated tumours, TSC patients displayed a reduced seizure frequency and improved memory function in addition to tumour shrinkage [49] , [50] . mTOR inhibitors may also benefit individuals who have other diseases in which TSC-mTOR signalling is involved [14] , [19] , [20] . Phenotypic amelioration of neural-specific Pten knockout mice [48] suggests that mTOR inhibitors may be feasible for the treatment of patients who carry PTEN mutations, constituting a substantial part of the genetic causes of ASD [6] , [8] . The altered mRNA expression of Mapk1 and Gsk3b in Tsc2 +/− mice may be related to dysregulated mTOR signalling observed in mouse models of neurofibromatosis type I [51] , [52] , [53] and FXS [54] , [55] . These two diseases are associated with neuropsychiatric complications, including ASD [6] , [14] , [19] , [20] , and mTOR inhibitors might be indicated. However, according to a recent publication, the hippocampus in Tsc2 +/− mice exhibited deficient long-term synaptic depression dependent on metabotropic glutamate receptor 5 (mGluR5) and decreased protein synthesis [56] , the opposite of exaggerated mGluR5-dependent long-term synaptic depression and protein synthesis observed in Fmr1 knockout mice [57] . Elevated mTOR activity is the primary cause of deficient social behaviour in TSC and PTEN mutations, whereas it may be a secondary change in FXS. Further investigations should elucidate the entire substrates that give rise to social deficits in these disorders that involve mTOR signalling. In conclusion, we found that Tsc1 +/− and Tsc2 +/− mice, both male and female, exhibited deficient social interaction. The deficit in adult heterozygotes was reversed by pharmacological inhibition of mTOR. We also demonstrated that the behavioural abnormality was associated with alterations of the mTOR signalling pathway at the mRNA and protein levels, which were rapamycin-sensitive. This indicates the pathogenetic role of aberrant mTOR signalling in social deficits and its reversible nature in Tsc1 +/− and Tsc2 +/− mice. The above findings are expected to encourage clinical trials of mTOR inhibitors as pharmacological treatments of ASD in individuals with TSC and possibly other disorders associated with dysregulated mTOR signalling. Mice Tsc1 +/− and Tsc2 +/− mice were generated as previously described [23] , [24] , and backcrossed to a C57BL/6J background for more than 10 generations. All of the mice were housed in groups of 2–6 per cage, segregated by sex, in a room on a 12 h/12 h light/dark cycle (lights on at 8:00 AM, off at 8:00 PM) maintained at 22±2 °C. All of the experiments were conducted blind to genotype and treatment and performed during the light cycle. The behavioural tests in the naive condition were performed at 8–10 weeks of age for open-field test, pole test and rotarod test. The remaining tests in the naive condition and all of the tests with rapamycin were conducted at 3–7 months of age. All of the animal experiments were performed in accordance with the Guidelines for the Care of Laboratory Animals of the Tokyo Metropolitan Institute of Medical Science, and the housing conditions were approved by the Institutional Animal Care and Use Committee. Rapamycin Rapamycin (LC Laboratories, Woburn, MA, USA) was dissolved in 10% dimethyl sulfoxide diluted with saline to 10 ml kg −1 . The mice received the rapamycin solution (2, 5 and 10 mg kg −1 ) or an equal volume of vehicle by intraperitoneal injection once daily for 2 consecutive days. The behavioural tests and brain collection were performed 24 h after the second administration. Social interaction test Each mouse was left alone in its home cage for 15 min. An unfamiliar C57BL/6J mouse of the same sex was then introduced. The behaviour of the test mouse was video-recorded for 10 min and scored for active interaction (that is, sniffing, allo-grooming, mounting and following) and rearing behaviour. Tube test for social dominance A pair of WT mice and an unfamiliar heterozygous mouse of the same strain and sex were placed into opposite ends of a clear plastic tube (33 cm length, 3.5 cm (male) and 2.6 cm (female) diameter). The side from which the heterozygote entered was assigned alternately. The test ended when one mouse completely retreated from the tube, and the remaining mouse was defined as the winner. The winners were analysed with regard to genotype, the side from which the winner entered, and differences in body weight that were >5%. Food exploration test Each mouse was deprived of food for 16 h before testing while water was freely available. The mouse was then placed in its home cage with one food pellet (0.5 g) buried 0.5 cm under the bedding material. The time required to find the food was measured by direct observation. Novel object test Each mouse was left alone in its home cage (32 × 21 × 13 cm) for 15 min. A white plastic bottle (6 cm diameter, 6 cm height) was then placed in the centre of the cage. The behaviour of the mouse was video-recorded for 10 min and analysed for exploration (that is, sniffing, touching or gnawing the bottle). Neurological examination and general condition Upon weaning at postnatal day 28–32, each mouse was observed for general appearance and neurological reflexes [58] . The mice were weighed at 6 weeks of age. Open-field test Each mouse was placed into a cylindrical open field (30 cm diameter, 30 cm height). Locomotor activity was counted using SuperMex (Muromachi Kikai, Tokyo, Japan) for 120 min. Pole test Each mouse was placed with its head facing upward on the top of a wooden pole (1 cm diameter, 50 cm height) vertically fixed to the floor. The mouse was first acclimated to the pole in three trials. Next day the mouse was allowed to descend five times in a single session. The latencies to reach the floor (that is, the time to descend) were measured, and the shortest latencies were kept. Rotarod test Each mouse was trained to run on a rotating rod (9 cm diameter, 10 rotations per minute; Muromachi Kikai, Tokyo, Japan) five times per day for 5 consecutive days. The longest latency to fall was recorded on each test day. Hot-plate test The mouse was placed on a heating apparatus (Muromachi Kikai, Tokyo, Japan) maintained at 52 °C. The time that elapsed until the mouse licked its hindpaw or jumped was measured by an experienced observer. The test was repeated three times at an interval of 15 min, and the median values were analysed. Tail flick test Each mouse was wrapped with black velvet, and its tail was heated (Muromachi Kikai, Tokyo, Japan). The latency to flick the tail was measured automatically. The median values of three measurements were collected. Tail suspension test Each mouse was suspended with adhesive tape so that its whiskers did not touch the floor. Immobility was detected automatically (MicroAct ver. 1.0, Neuroscience, Tokyo, Japan) for 6 min. Light/dark box test. The test apparatus consisted of a plastic box (35 × 15 × 17 cm) divided into two compartments of equal size, separated by two small openings. One chamber was white and brightly lit (580 lux), and the other was black and kept dark. Each mouse was placed into the light compartment and allowed to move freely for 10 min. The time spent staying in the dark chamber was measured automatically (Neuroscience, Tokyo, Japan). Whole-genome expression analysis Total RNA was isolated from whole brain using Sepasol-RNA I Super solution (Nacalai Tesque, Kyoto, Japan), and the extracted RNAs (50 ng) were amplified with the TargetAmp Nano-g Biotin-aRNA Labelling Kit (Epicentre Biotechnologies, Madison, WI, USA). First-strand cDNA was synthesized from total RNA with T7-oligo (dT) primer, and second-strand cDNA synthesis was then performed with the first-strand cDNA. The in vitro transcription reaction was performed with the product of the second-strand cDNA synthesis to produce biotin-cRNAs by incorporating biotin-UTP into the RNA transcripts. Biotin-cRNA (750 ng) was further hybridized with MouseRef-8 Expression BeadChips (Illumina, San Diego, CA, USA) and then reacted with streptavidin-Cy3. The expression intensities of the transcripts on the BeadChips were detected by an Illumina iScan reader (Illumina, San Diego, CA, USA) as values above the internal standard. Quantitative real-time PCR analysis Quantitative real-time PCR analysis was performed using a LightCycler 480 II system (Roche Diagnostics Japan, Tokyo, Japan). The cDNAs were reverse-transcribed from total RNAs isolated from whole brains with the SuperScript III First-Strand Synthesis System for real-time PCR according to the manufacturer’s instructions (Invitrogen Life Technologies Japan, Tokyo, Japan). The specific primers and hybridization probes (Universal ProbeLibrary Probes) for real-time PCR were designed using a web-based platform, Universal ProbeLibrary Assay Design Center (Roche Diagnostics Japan; Supplementary Table S6 ). Real-time PCR was performed with a LightCycler 480 Probes Master, specific primers and Universal ProbeLibrary probes. The PCR thermal cycle conditions were the following: 95 °C for 5 min (denature); 45 cycles at 95 °C for 10 s, 60 °C for 30 s and 72 °C for 1 s (amplification); 95 °C for 10 s, 50 °C for 30 s and up to 70 °C (ramping rate, 0.06 °C s −1 ; melting curve). PCR was performed in duplicate wells for each target transcript and sample, and the relative expression of target transcripts, calculated using the comparative C T method with the second derivative maximum procedure, was normalized to that of β-actin mRNA. Antibodies A rabbit anti-mouse hamartin polyclonal antibody (TSC1/Hamartin(T1146), 1.5 μg ml −1 ) was produced by immunization with a synthetic peptide that consisted of a carboxy-terminal sequence (GQLHIMDYNETHPEHS) and cysteine residue for conjugation and purified by antigen peptide affinity chromatography (Immuno-Biological Laboratories, Gunma, Japan). Rabbit anti-tuberin (1 μg ml −1 ), anti-actin (0.4 μg ml −1 ) and anti-S6K (0.4 μg ml −1 ) antibodies were purchased from Santa Cruz Biotechnology (Santa Cruz, CA, USA). Rabbit anti-phospho-Akt (S473) (1:500), anti-Akt (1:500), and anti-phospho-S6K (T389) (1:500) antibodies were purchased from Cell Signaling Technology (Danvers, MA, USA). Western blotting Whole brains were homogenized by a tissue homogenizer in 1 × SDS gel-loading buffer (50 mM Tris–HCl at pH 6.8, 2% SDS and 10% glycerol). The supernatant was obtained by centrifugation, and the protein concentration was determined using the Bio-Rad DC Protein Assay Kit (Bio-Rad Laboratories, Hercules, CA, USA). Equal amounts of protein extracted were added with 5% mercaptoethanol and boiled. Proteins were resolved by SDS–PAGE, transferred onto a polyvinylidene fluoride membrane (Immobilon-P, Merck Millipore, Billerica, MA, USA) and blocked in 1% skim milk/Tris-buffered saline that contained 0.05% Tween 20 at room temperature for 2 h. The membranes were incubated with the primary antibodies at room temperature for 1 h. Protein bands were detected using the EnVision+ Kit (Dako, Glostrup, Denmark) and ECL Western Blotting Detection System (GE Healthcare, Buckinghamshire, UK) and quantitatively analysed using ImageJ software (ver. 1.45). The values of each protein were normalized to that of actin. Statistical analysis The statistical analyses were conducted with StatView ver. 5.0 software (SAS Institute). Data were analysed using a two-tailed t -test, one-way ANOVA followed by Dunette post hoc test, two-way ANOVA, and three-way mixed design ANOVA as noted in the test. A binominal test was used for the tube test. Data from the rapamycin experiments were pooled with regard to sex before the statistical analysis. Values of P <0.05 were considered statistically significant. How to cite this article: Sato, A. et al. Rapamycin reverses impaired social interaction in mouse models of tuberous sclerosis complex. Nat. Commun. 3:1292 doi: 10.1038/ncomms2295 (2012).